A pairwise maximum entropy model accurately describes resting-state human brain networks The resting-state human brain networks underlie fundamental cognitive functions and consist of complex interactions among brain regions. However, the level of complexity of the resting-state networks has not been quantified, which has prevented comprehensive descriptions of the brain activity as an integrative system. Here, we address this issue by demonstrating that a pairwise maximum entropy model, which takes into account region-specific activity rates and pairwise interactions, can be robustly and accurately fitted to resting-state human brain activities obtained by functional magnetic resonance imaging. Furthermore, to validate the approximation of the resting-state networks by the pairwise maximum entropy model, we show that the functional interactions estimated by the pairwise maximum entropy model reflect anatomical connexions more accurately than the conventional functional connectivity method. These findings indicate that a relatively simple statistical model not only captures the structure of the resting-state networks but also provides a possible method to derive physiological information about various large-scale brain networks. During rest, the human brain is not idle but shows a large amount of spontaneously fluctuating activity that is highly correlated between multiple brain regions [1] , [2] . Previous studies used positron emission tomography or functional magnetic resonance imaging (fMRI) to reveal that brain regions interact with each other during rest and constitute several resting-state networks (RSNs) [3] , [4] , [5] , [6] . The RSNs, including the default mode network (DMN) [5] , [6] and the fronto-parietal network (FPN) [7] , [8] , are highly reproducible across different healthy individuals [9] and are considered to underlie fundamental and intrinsic functions such as self-referential cognitive processes [10] , [11] , maintenance of memory [12] and attentional cognitive processes [8] . These functions are considered to originate from complex functional interactions among the brain regions belonging to the RSNs [13] . However, the level of complexity that is observed in the activities of an ensemble of brain regions and in the structure of these functional interactions has not been quantified for the RSNs. As a result, it remains challenging to comprehensively understand this ensemble brain activity as an integrative large-scale neural system [14] , [15] . For microscopic neural tissues, maximum entropy models (MEMs) have been successful in estimating the complexity of neural activity patterns. For example, the pairwise MEM method (that is, a second-order model) seeks to fit a relatively simple binary-state model containing up to second-order interaction terms (that is, firing rates and pairwise interaction) to empirical data of spatiotemporal spike trains. If the pairwise MEM is accurately fitted to the data, activity patterns of neurons can be described with a combination of averaged activity at each recording site and pairwise correlation. If it does not, we cannot ignore higher-order interactions such as triplet interactions originating from an external common input, and accurate descriptions of the activity patterns of neurons would require more complicated (that is, higher-order) MEM models. In fact, the pairwise MEM accurately describes firing patterns in the retinal tissues of primates recorded electrophysiologically in vitro [16] , [17] , [18] , [19] , [20] , [21] , firing patterns and local field potentials (LFPs) in human cortical tissues in vitro [22] and large-scale firing patterns in the visual cortex of monkeys and cats in vivo [23] , [24] . These findings suggest the possibility that the human brain activity patterns during rest are not so complex and can be accurately described by pairwise MEMs. If the pairwise MEM accurately explains large-scale brain activity patterns during rest, the MEM method will give us much richer information about functional interactions in the RSNs than the widely used functional connectivity (FC) analysis, which is based on Pearson’s correlation coefficient between a pair of brain regions. Although FC often implies broader classes of methods for inferring connectivity in the brain, we use this term to refer to the methods on the basis of Pearson’s correlation coefficient in this paper. The FC-based analysis (based on Pearson’s correlation coefficient) has successfully revealed that specific functional connexions are enhanced during specific cognitive processes [25] , [26] , and the FC map serves as a promising indicator of several diseases [27] , [28] , stages of development [29] , [30] and levels of intelligence [31] . However, because FC is calculated as Pearson’s correlation coefficient between activities of pairs of regions [3] , [4] , the FC-based method is founded on the implicit assumption that the pairwise interactions are independent of each other [32] . If different pairwise interactions influence each other, the observed correlation between regions A and B may be a natural consequence of, for example, the correlation between regions A and C and that between regions B and C. In fact, a study employing monkeys shows that, even when a pair of brain regions does not have a direct anatomical connexion, the FC between them is often large if the regions receive common input from a third region [33] . Other studies also show that a significant FC value between a pair of regions does not distinguish a direct (that is, monosynaptic) connexion from an indirect (that is, polysynaptic) connexion [34] , [35] . The FC-based methods may discard possibly rich information that would be revealed if we take into account that functional interactions influence each other [8] . Unlike the functional interactions estimated by the FC-based method, functional interactions estimated by the pairwise MEM method are not a simple collection of pairwise interactions that are determined independently of each other. The method infers organization of functional interactions based on global activity patterns (that is, activities of more than two sites that are considered simultaneously), not on the assumption that activity patterns of region pairs are independent of those of other pairs. Therefore, if the pairwise MEM can accurately describe the RSNs, the MEM method is expected to provide a better method for assessing integrative network structure than the FC-based method. In the present study, we first quantify the complexity inherent in activities of an ensemble of brain regions during rest by fitting the MEM to resting-state fMRI data in the RSNs. Then, to validate the approximation of the RSNs by the pairwise MEM, we demonstrate that the interactions estimated by the pairwise MEM are more physiologically informative than those estimated by FC in the sense that anatomical connexions are more accurately predicted. The pairwise MEM even outperforms other methods that take into account global activity patterns beyond a collection of independently estimated pairwise interactions, including the partial correlation method [36] , [37] and the mutual information (MI) method [37] , [38] , [39] . Acquisition and processing of data We applied the pairwise MEM to fMRI signals obtained from the brain regions belonging to the DMN [5] , [6] and FPN [7] , [8] , two representative RSNs. We separately applied the pairwise MEM to the DMN and FPN, which are relatively independent of each other in the sense that they are thought to have different functions [15] , [40] . The coordinates of the brain regions were anatomically defined based on a meta-analysis of resting-state fMRI data obtained from 183 healthy participants [41] , [42] . 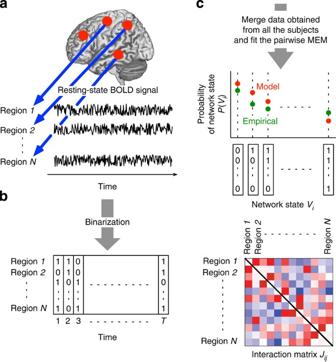Figure 1: Fitting the pairwise MEM to fMRI data. (a,b) Resting-state BOLD signals are extracted from anatomically defined regions (a) and binarized (b). (c) If the pairwise MEM is accurately fitted to the binarized data, the estimated probability distribution of the network state will resemble the empirical distribution (top). The pairwise MEM also provides an interaction matrix (bottom). The DMN and FPN consisted of 12 and 11 regions, respectively ( Table 1 ). We obtained ∼ 45 h of resting-state fMRI data from six healthy young adult participants ( ∼ 7.5 h per participant). Using the data, we extracted the low-frequency signals (0.01–0.1 Hz) from all the brain regions included in the DMN or FPN ( Fig. 1a ), binarized the signals ( Fig. 1b ) and fitted the MEM to the binarized signals ( Fig. 1c ). Table 1 Coordinates of brain regions in the RSNs. Full size table Figure 1: Fitting the pairwise MEM to fMRI data. ( a , b ) Resting-state BOLD signals are extracted from anatomically defined regions ( a ) and binarized ( b ). ( c ) If the pairwise MEM is accurately fitted to the binarized data, the estimated probability distribution of the network state will resemble the empirical distribution (top). The pairwise MEM also provides an interaction matrix (bottom). Full size image Accurate fitting of the pairwise MEM to resting-state fMRI signals In Fig. 2a , each data point represents the estimated and empirical probabilities that a binarized activity pattern (that is, state vector in Fig. 1c ) occurs. If the points are on the diagonal (lines in Fig. 2a ), the model would perfectly explain the empirical activity patterns. For comparison, the results for the MEM estimated under the restriction that different regions do not interact (that is, independent MEM) are also presented in the figures. 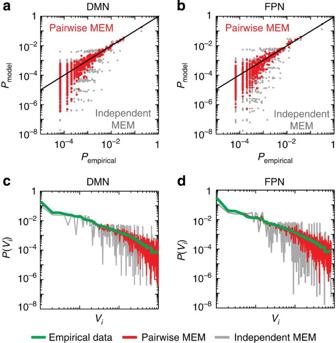Figure 2: Accurate fitting of the pairwise MEM. (a,b) Comparison between the probabilities of network states for empirical data and those estimated for the pairwise and independent MEMs. The red and grey dots indicate the results for the pairwise and independent MEMs, respectively. (c,d) The probability of a network state for the MEMs,P(Vi), is plotted against the network state, (Vi). The network states are shown in descending order of empirical probability. The red and grey lines represent the results for the pairwise and independent MEMs, respectively. The green lines represent the empirical data. Figure 2a suggests that, in both the DMN and FPN, the pairwise MEM explains the empirical frequency of the activity patterns much more accurately than the independent MEM. In both the DMN and FPN, the probability of the pattern estimated by the pairwise MEM was generally closer to the empirical probability than that estimated by the independent MEM for both rare and frequent patterns ( Fig. 2c ). The pairwise MEM results in a high accuracy (85% for the DMN and 94% for the FPN). An accuracy of 85%, for example, indicates that the application of the pairwise MEM reduces the distance between the estimated and empirical distributions of patterns by 85% as compared with the independent MEM (see equation (2) in the Methods ). These results show that the pairwise MEM accurately describes the fMRI signals in the RSNs. Figure 2: Accurate fitting of the pairwise MEM. ( a , b ) Comparison between the probabilities of network states for empirical data and those estimated for the pairwise and independent MEMs. The red and grey dots indicate the results for the pairwise and independent MEMs, respectively. ( c , d ) The probability of a network state for the MEMs, P ( V i ), is plotted against the network state, ( V i ). The network states are shown in descending order of empirical probability. The red and grey lines represent the results for the pairwise and independent MEMs, respectively. The green lines represent the empirical data. Full size image Robustness of accurate fitting of the pairwise MEM We then examined the robustness of the accurate fitting of the pairwise MEM from three perspectives. First, we evaluated the accuracy of fit for various values of the threshold for binarization, because the pairwise MEM requires binarization of the originally continuous fMRI signals ( Fig. 1b ). 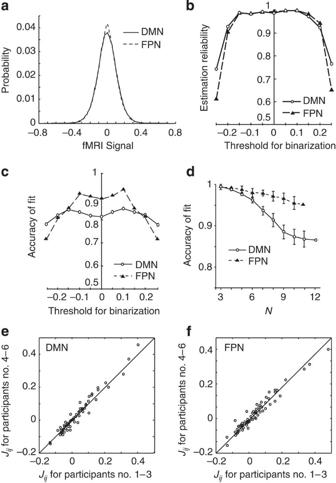Figure 3: Robustness of fitting. In panels (a–d) solid and dashed lines represent the results for the DMN and FPN, respectively. (a) Distributions of the preprocessed resting-state fMRI signals. (b) Relationships between the estimation reliability for the pairwise MEM (equation (3)) and the threshold for binarization. (c) Relationships between the accuracy of fitting for the pairwise MEM (equation (2)) and the threshold for binarization. (d) Dependence of the accuracy of the fitting for the pairwise MEM on the number of regions. Symbols:average, Error bar: s.d. For example, there are 220 different sub-networks (combinations) ofN=3 regions for the DMN. (e,f) Scattergrams of the interaction weights obtained from the pairwise MEM fitted to the data for participants no. 1–3 and those obtained from participants no. 4–6 show that the results do not vary by subject. The distributions of the original continuous signals for the two RSNs are shown in Figure 3a . We then set various threshold values for binarization within the range of the fMRI signal, and tested the dependence of the so-called estimation reliability on the threshold. The estimation reliability represents the precision with which the parameters in the pairwise MEM are estimated (see equation (3) in the Methods ). The pairwise MEM estimated the parameter values with high reliability (>99%) when the threshold lay approximately between −0.15 and 0.15 ( Fig. 3b ). Consistent with this result, the fitting of the pairwise MEM to the data was accurate for threshold values in this range (>80% for the DMN and >90% for the FPN; Fig. 3c ). The threshold of −0.15, for example, implies that the accuracy of fit remains high even if the probabilities of the two binarized states of a brain region are quite uneven (that is, activated with probability 0.78 and not activated with probability 0.22). These results suggest that the accuracy of fit is robust as long as the threshold is located between −0.15 to 0.15. In the following, we set the threshold to 0.1 because this value maximized the accuracy of fit of the pairwise MEM ( Fig. 3c ). Figure 3: Robustness of fitting. In panels ( a – d ) solid and dashed lines represent the results for the DMN and FPN, respectively. ( a ) Distributions of the preprocessed resting-state fMRI signals. ( b ) Relationships between the estimation reliability for the pairwise MEM (equation (3)) and the threshold for binarization. ( c ) Relationships between the accuracy of fitting for the pairwise MEM (equation (2)) and the threshold for binarization. ( d ) Dependence of the accuracy of the fitting for the pairwise MEM on the number of regions. Symbols:average, Error bar: s.d. For example, there are 220 different sub-networks (combinations) of N =3 regions for the DMN. ( e , f ) Scattergrams of the interaction weights obtained from the pairwise MEM fitted to the data for participants no. 1–3 and those obtained from participants no. 4–6 show that the results do not vary by subject. Full size image Second, we confirmed that the high accuracy of our results was not due to a fallacy of the pairwise MEM when it is applied to too small populations. When the accuracy of the fitting linearly decreases with the number of regions N , one theory suggests that the accurate fitting may be an artifact of a small N [43] . In this case, the validity of the pairwise MEM cannot be directly extrapolated to populations with a large N [43] . For our data, the accuracy decreases sub-linearly with N at least for the DMN ( Fig. 3d ). Furthermore, the theory indicates that the pairwise MEM can be informative about empirical data only when it is accurately fitted to data with N significantly larger than , where and δt are the averaged activation rate and the length of the time bin, respectively [43] . In the present analysis, =0.045 s −1 and =0.041 s −1 for the DMN and FPN, respectively, and δt =9.045 s. Therefore, N c ≈2.5 and 2.7 for the DMN and FPN, respectively. Figure 3d suggests that the pairwise MEM was accurate for the two networks up to N =12 and 11, which are much larger than N c . Therefore, the high accuracy of the pairwise MEM for our data is not an artifact of a small N value. Third, we examined the dependence of the results on the participants. We split the fMRI data into two groups, that is, the data obtained from participants no. 1–3 and those obtained from participants no. 4–6. The interaction weights (that is, elements of the estimated interaction matrix, denoted by J ij in equation (1); also see Fig. 1c ) obtained from the pairwise MEM were similar between the two groups (Pearson’s correlation coefficient r =0.96, P <10 −3 in Fig. 3e ; r =0.93, P <10 −3 in Fig. 3f ). Therefore, our results are robust with respect to the participants. In summary, the pairwise MEM accurately and robustly explains the collective activities of the brain regions in the RSNs. Interaction matrices derived by the pairwise MEM and alternative methods If the functional interactions estimated by the pairwise MEM are closely relevant to some physiological basis, the relationship would provide further validation of the approximation of the RSNs by the pairwise MEM. Therefore, we next examined the possible physiological bases of the interaction weights between pairs of regions inferred by the pairwise MEM. For comparison, we referred to large-scale anatomical connectivity determined from previous diffusion tensor imaging (DTI) of the brains of 80 healthy young human adults [44] . To assess the performance of the pairwise MEM, we also generated four types of interaction matrices as controls, that is, those based on the FC method, those based on the inverse Gaussian model, those based on the partial correlation method [36] , [37] and those based on the MI method [37] , [39] (see Methods ). It should be noted that the four methods do not require binarization of the fMRI signals. The anatomical connectivity maps and the interaction matrices estimated by the five methods are shown in Fig. 4 . For both the DMN ( Fig. 4a ) and FPN ( Fig. 4b ), the | J ij | values estimated by the pairwise MEM are mainly large for pairs of brain regions with direct anatomical connexion, whereas, in the other methods, | J ij | is large both for pairs with direct anatomical connexion and those without such connexion. Therefore, the pairwise MEM seems to outperform the other four methods in estimating the anatomical connexions if we regard both positive and negative large values of J ij as predicting the presence of anatomical connexion. The use of both positive and negative values is consistent with the anatomical evidence, because anatomical results derived from DTI are thought to reflect either excitatory or inhibitory connectivity between pairs of regions. 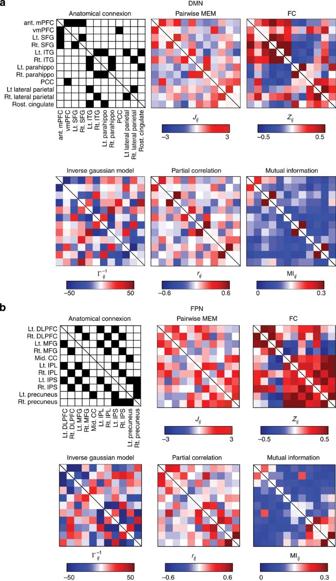Figure 4: Anatomical connexions and interaction matrices. (a,b) Upper left panels show anatomical connexion maps. The other panels show the interaction matrices based on the pairwise MEM, FC, inverse Gaussian model, partial correlation method and MI method. The abbreviations of the regions are explained inTable 1. Figure 4: Anatomical connexions and interaction matrices. ( a , b ) Upper left panels show anatomical connexion maps. The other panels show the interaction matrices based on the pairwise MEM, FC, inverse Gaussian model, partial correlation method and MI method. The abbreviations of the regions are explained in Table 1 . Full size image Prediction of anatomical connexions by the pairwise MEM and the other methods To analyse the results more quantitatively, we compared the accuracy of the five methods in estimating the presence or absence of the anatomical connexions between pairs of regions. 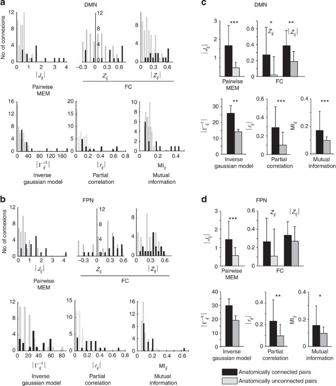Figure 5: Statistical comparison of interaction matrices with anatomical connexions. In all the panels, the black and grey bars indicate the results for the anatomically connected pairs and anatomically unconnected pairs, respectively. (a,b) Histograms of the interaction weights for anatomically connected and unconnected pairs. (c,d) Comparison of the average interaction weight between anatomically connected and unconnected pairs. Error bars: s.d., ***P<0.005, **P<0.01, *P<0.05, in two-samplet-tests. Figure 5a shows histograms of the values of interaction weights (that is, values of the entries of the matrices shown in Fig. 4 ) estimated by the five methods. As the absolute value of the functional interaction weight seems to predict the anatomical connexions better than the raw values of them, at least for all the methods except FC, we show the histograms of the absolute values of the interaction weights. However, for the FC, we also show the histograms of the raw values of the interaction weights (that is, correlation coefficient) because they are conventionally used [34] , [41] , [45] . Figure 5: Statistical comparison of interaction matrices with anatomical connexions. In all the panels, the black and grey bars indicate the results for the anatomically connected pairs and anatomically unconnected pairs, respectively. ( a , b ) Histograms of the interaction weights for anatomically connected and unconnected pairs. ( c , d ) Comparison of the average interaction weight between anatomically connected and unconnected pairs. Error bars: s.d., *** P <0.005, ** P <0.01, * P <0.05, in two-sample t -tests. Full size image Under the pairwise MEM, anatomically connected pairs of regions in both the DMN and FPN tended to have larger absolute values of interaction weights than pairs that were not directly connected in anatomy. The interaction weights for the anatomically connected pairs were significantly larger than those for the anatomically unconnected pairs on average ( P <0.001, two-sample t -tests in both the DMN and FPN; Fig. 5c ). The partial correlation and MI methods yielded similar significant differences between the anatomically connected pairs and unconnected pairs (for both models, P <0.001 in DMN, P <0.05 in FPN, two-sample t -tests; Fig. 5c . Also see Fig. 5a ). In contrast, the FC and inverse Gaussian models did not predict anatomical connexions as accurately as the pairwise MEM ( Fig. 5a ). In the DMN, the interaction weights estimated by these two methods had larger values when region pairs were anatomically connected than unconnected (FC: P <0.05, absolute value of FC: P <0.01, inverse Gaussian model: P <0.01, two-sample t -tests). However, in the FPN, the difference was insignificant for both of the two methods ( P >0.3). For further comparison the five methods, we carried out a receiver-operating characteristic (ROC) analysis, which is sensitive to the difference in the distribution of the functional interactions between the anatomically connected and unconnected pairs ( Fig. 6a ). In short, the curves show the relationship between the false positive (that is, anatomically unconnected pairs whose interaction weights exceed a threshold) and true positive (that is, anatomically connected pairs whose interaction weights exceed the same threshold; also called the sensitivity) when we vary the threshold for classifying the region pairs into anatomically connected and unconnected groups. When the false positive is small and the true positive is large for a threshold value, the classification is accurate such that the interaction weights determined by an estimation method are relatively consistent with the anatomy. In both the DMN and FPN, the area under the curve (AUC) for the pairwise MEM was significantly larger than those for the other four methods (DMN: Z >7.3, P <1.0 × 10 −11 , Bonferroni-corrected; FPN: Z >9.4, P <1.0 × 10 −16 , Bonferroni-corrected; Fig. 6c ). There was no significant difference between any other pair of the methods. 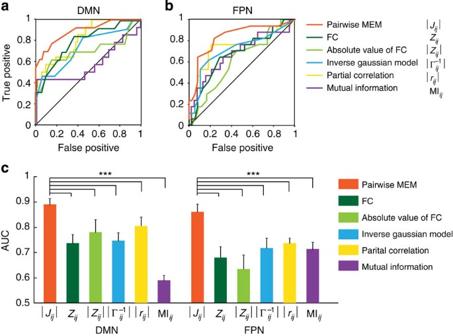Figure 6: ROC analysis. The colour code is as follows: red, pairwise MEM; green, raw values of FC; light green, absolute values of FC; blue, inverse Gaussian model; yellow, partial correlation method; purple, MI method. (a,b) ROC curves for the classification into anatomically connected and unconnected region pairs based on the interaction weights. (c) AUCs of the ROC curves shown in panels (a,b). Error bars: s.d., ***P<0.005, in two-samplet-tests with the Bonferroni correction. Figure 6: ROC analysis. The colour code is as follows: red, pairwise MEM; green, raw values of FC; light green, absolute values of FC; blue, inverse Gaussian model; yellow, partial correlation method; purple, MI method. ( a , b ) ROC curves for the classification into anatomically connected and unconnected region pairs based on the interaction weights. ( c ) AUCs of the ROC curves shown in panels ( a , b ). Error bars: s.d., *** P <0.005, in two-sample t -tests with the Bonferroni correction. Full size image Validity of binarizing fMRI signals We binarized the fMRI signals to implement the pairwise MEM. However, fMRI signals originally represent continuous blood flows to brain regions, and the validity of the binarization is unclear. Therefore, we calculated the accuracy of fit of pairwise MEMs in which the signals were classified to three discrete levels, which we call the trinary MEM, by using a standard procedure described in Methods [46] . When the signals recorded at the different brain regions and time points were evenly divided into three groups ( Supplementary Fig. S1 ), the accuracy of fit was the highest. However, the accuracy of fit in this case was approximately equal to 0.55 ( Supplementary Fig. S2 ) and significantly lower than those obtained for the binary pairwise MEM for both the DMN and FPN ( P <10 −3 in two-sample t -tests). Despite the lower accuracy of the trinary MEM, the trinary MEM might be better at accurately predicting anatomical connectivity than the binary MEM. Therefore, we examined the relationship between the functional interactions estimated by the trinary MEM and the anatomical connectivity. For the trinary MEM, the functional interactions between anatomically connected pairs were larger than those between anatomically unconnected pairs ( P <0.05 in two-sample t -tests, Supplementary Fig. S3 ). However, ROC analysis revealed that the AUC for the trinary MEM was significantly smaller than that for the binary MEM ( P <10 −3 in two-sample t -tests, Supplementary Fig. S4 ). These results suggest that the binary pairwise MEM provides more information about anatomical connectivity than the trinary pairwise MEM. Such a difference usually arises because the trinary MEM requires a larger amount of data than the binary MEM (that is, 3 N versus 2 N data points). However, even the trinary MEM with N =4 and N =5, for which there are relatively few activity patterns (that is, 3 4 =81 and 3 5 =243 patterns), yields the accuracy of fit values <0.6. These accuracy of fit values are much smaller than those for the binary MEM with comparable numbers of activity patterns: the accuracy of fit was >0.9 for the binary MEM with N =8, with which there are 2 8 =256 activity patterns ( Fig. 3d ). Therefore, we conclude that the binary MEM better captures fMRI signals than the trinary MEM and presumably MEMs that allow more discrete levels. We have demonstrated that the pairwise MEM accurately describes activity in the human RSNs. The model was fitted to both the DMN and the FPN with high accuracy and robustness. Furthermore, functional interaction matrices derived from the pairwise MEM were similar to the anatomical connexion maps. The agreement between the estimated matrices of functional interactions and the anatomical maps is better with the pairwise MEM than with the four other methods: the FC based on Pearson’s correlation coefficients, inverse Gaussian model, partial correlation method and MI method. These findings suggest that the large-scale human brain networks during rest can be captured by a relatively simple second-order model. Our results extend the previous findings that the pairwise MEM accurately describes activity patterns observed in a slice or small parts of the brain [16] , [17] , [18] , [19] , [22] , [23] , [24] . In particular, Tang and colleagues [22] showed that the pairwise MEM approximates the statistics of multiunit LFPs recorded from cultured slices of the human brain cortex. As LFPs are considered to be predictive of blood-oxygenation-level-dependent signals (that is, fMRI signals) [47] , it is reasonable that the present study has successfully fitted the pairwise MEM to fMRI signals. Although fine-scale neural networks (<300 μm) seem to require more complex models, such as higher-order MEMs [19] , [24] , in terms of the spatial scale, we have extended the applicability of the pairwise MEM method from microscopic neural populations ( ∼ 500 μm) to macroscopic populations at the level of the entire brain ( ∼ 10 cm). In previous studies, large FC values have been suggested to imply the presence of direct anatomical connexion between regions [2] , [34] , [45] . In particular, a study using high-resolution fMRI conducted an ROC analysis similar to ours, and reported that the FC classifies the anatomical connexions with high accuracy (AUC=0.79) [34] . Our present study produced similar accuracy values for the FC (AUCs in the DMN and FPN of 0.73 and 0.67, respectively; Fig. 6c ) but also showed that the pairwise MEM gives higher accuracy (AUC in the DMN and FPN of 0.89 and 0.85, respectively; Fig. 6c ). These results suggest that the pairwise MEM captures the anatomical properties of large-scale brain networks to a better extent than the FC-based method does, although the pairwise MEM is a statistical model and not based on the physiology of the brain. As second-order interaction implies networks consisting of nodes and links, the pairwise MEM may serve as a tool for investigating large-scale human brain networks. As previous studies did for networks generated by the resting-state FC (see a review [14] ), we can in principle calculate various graph-theoretical quantities for the RSNs defined by the pairwise MEM. This approach calls for a sufficient amount of resting-state fMRI data to estimate an interaction matrix among a relatively large number of brain regions and efficient algorithms to estimate the MEM for large N , such as those developed in previous studies [19] , [48] , [49] . We can also apply the pairwise MEM to fMRI data measured during psychological tasks, though several modifications of the method may be in order. In previous fMRI studies, such task-specific functional interactions were estimated by psychophysiological interaction analysis [50] , Granger causality analysis [51] and dynamic causal modelling [52] . Among these methods, psychophysiological interaction analysis, like FC-based methods, is a seed-based analysis and does not allow us to collectively estimate functional interactions among the entire set of recorded sites. The use of dynamic causal modelling and Granger causality modelling still seems to be limited [8] , [53] . Therefore, the pairwise MEM may serve as an alternative method for inferring task-specific brain networks. In particular, recent theoretical developments of the MEM incorporate causality (signal flow from one region to another) [54] , [55] , which will be an indispensable component for modelling task-related data. Participants and fMRI data acquisition Six healthy right-handed subjects (aged 20–23 years; three males) participated in the experiments after written informed consent was obtained. The MRI scanning was conducted using a 3T MRI scanner (Philips Achieva X 3T Rel. 2.6, Best, The Netherland). T1-weighted structural images were obtained for anatomical reference (resolution=0.81 × 0.81 × 1.20 mm 3 ). Functional imaging used gradient-echo echo-planar sequences (TR=9.045 s, TE=35 ms, flip angle=90°, resolution=2 × 2 × 2 mm 3 , 75 slices). The entire procedure for the MRI scanning was approved by the institutional review board of The University of Tokyo School of Medicine. During the functional imaging, the participants were instructed to passively view a fixation point on the screen. One passive fixation session took ∼ 5 min, and each participant underwent 90 sessions ( ∼ 7.5 h) on 6–8 separate days. In each session, we discarded the first five images (9.045 s/volume × 5 volumes=45.225 s) to exclude the influence of transient processes before the equilibrium of longitudinal magnetization. In total, 17,820 volumes (2,970 volumes per participant) of resting-state functional images were obtained. Preprocessing of fMRI data In line with previous studies of resting-state fMRI [25] , [26] , [30] , we preprocessed the fMRI data as follows. First, for each session and each participant, the functional images were realigned, their slice-timing was corrected and they were normalized to the standard template image (ICBM 152) by SPM8 ( www.fil.ion.ucl.ac.uk/spm/ ). Second, for each session, after temporal band-pass filtering (0.01–0.1 Hz) with Matlab scripts written in-house, the data underwent spatial smoothing (FWHM=8 mm) in SPM8. Third, the smoothed data originating from all the sessions were combined for each participant. Finally, for each participant, the combined data were corrected for their head motion, whole-brain signals, ventricular signals, white matter signals and run effect. Therefore, the fMRI signals used in our analysis have the same unit as that of the so-called ‘beta-value’ [56] , [57] , [58] except for a normalization factor. We determined the coordinates of the brain regions belonging to the DMN and FPN based on a previous meta-analysis of resting-state fMRI studies [30] , [42] (the DMN: 12 regions, the FPN: 11 regions, Table 1 ). We subjected the preprocessed data corresponding to these brain regions to the following analysis. Pairwise MEM We fit the pairwise MEM to the resting-state fMRI data in essentially the same manner as did the previous studies of microscopic neural activities [16] , [17] , [22] , [23] , [24] . We added a constant to the preprocessed signal at each region such that the average of the preprocessed signals over T =17,820 snapshots (that is, functional images) is equal to zero at each region. Then the signals were binarized, because the pairwise MEM deals with snapshots of binarized signals recorded simultaneously at multiple sites. We set the bin width to 9.045 s, that is, one whole-brain image was taken in one repetition time (TR) of 9.045 s, because a long bin width is effective at decorrelating data that were recorded in adjacent time points. With a small bin width, the fMRI signals (that is, network states) in close time points would be highly correlated with each other. Therefore, the use of such a small bin width would not increase the effective number of samples. We experimented with various threshold values for binarization, and chose a value of 0.1, because it maximized the accuracy of fit ( Fig. 3b ). The binarized activity of brain region i at discrete time t , denoted by σ i t , is either on (+1) or off (0). The network state (that is, pattern) at time t is given in vector form by where N is the number of the brain regions of interest (that is, N =12 in the DMN and N =11 in the FPN). It should be noted that there are 2 N possible network states. The empirical activation rate of region i , denoted by 〈 σ i 〉, is given by . The empirical pairwise joint activation rate of regions i and j , denoted by 〈 σ i σ j 〉, is given by . The pairwise MEM maximizes the entropy of the distribution of activity patterns under the restriction that 〈 σ i 〉 and 〈 σ i σ j 〉 (1≤ i ≤ j ≤ N ) are preserved. It is known that such a distribution has the form , where P ( V i ) is the probability of network state V i , and h i represents the tendency of activation at region i , and J ij , called the interaction weight, represents functional interaction between regions i and j . Positive and negative values of J ij are interpreted as excitatory and inhibitory interactions, respectively. For an estimated probability distribution, the expected activation rate, 〈 σ i 〉 m , and the expected pairwise joint activation rate, 〈 σ i σ j 〉 m , are given by and , respectively, where σ i ( V j ) indicates the activity (either +1 or 0) of σ i under network state V j . We calculated h i and J ij by iteratively adjusting 〈 σ i 〉 m and 〈 σ i σ j 〉 m toward 〈 σ i 〉 and 〈 σ i σ j 〉, respectively, by using a gradient ascent algorithm. The iteration scheme is given by and , where α is the learning rate. We set α =0.75 to reduce computation time. We confirmed that the results were robust with respect to the choice of α ranging from 0.1 to 1.0. As in previous studies [16] , [17] , [22] , [23] , [24] , we evaluated the effectiveness of the pairwise MEM by using two information theoretic quantities. To define them, we also obtained the MEM without pairwise interaction between regions (that is, independent MEM) by determining h i (1≤ i ≤ N ) under the condition that J ij =0 (1≤ i , j ≤ N ). For the independent MEM, 〈 σ i σ j 〉 m is equal to 〈 σ i 〉 m 〈 σ j 〉 m . Using the resultant goodness of fit obtained for the two types of the MEMs, we define the accuracy index for the pairwise MEM by where is the Kullback–Leibler divergence between the probability distribution of the network state in the k th order model ( k =1 and 2 for the independent and pairwise MEMs, respectively) and the empirical distribution of the network state, denoted by P N . To evaluate reliability of the fitting, we calculate r S =( S 1 − S 2 )/( S 1 − S N ), where is the entropy of the distribution of the network state in the k th order model. Note that S N is the entropy of the empirical data. Using r S , we define the estimation reliability by The estimation reliability is equal to 1 if the values of h i and J ij are estimated without error [59] . Cross validation As a large sample size is desirable for statistical fitting, we trained the pairwise MEM using the entire data and tested it against the same data. To exclude the possibility of over fitting, we carried out cross validation as follows: (i) We divided the T observed snapshots (that is, network states) into the two subsets of equal size, that is, T /2, such that each snapshot independently belongs to either subset with probability 1/2. It should be noted that we are not concerned with the temporal structure of the data. (ii) We calculated the accuracy of fit by training the MEM using one subset and testing the estimated model against the other subset. (iii) We calculated the accuracy of fit by using one of the two subsets for both training and testing. (iv) We repeated procedures (i), (ii) and (iii) ten times and compared the accuracy of fit between the cross validation case (that is, (ii)) and the dependent training-testing case (that is, (iii)). We did not find significant differences between the two cases (cross validation versus dependent training-test cases: 0.67±0.0068 versus 0.68±0.0058 for the DMN, P >0.41; 0.76±0.0071 versus 0.76±0.0051 for the FPN, P >0.35, mean±s.d. in paired t -tests). Therefore, we concluded that the use of the same data in both training and testing did not give rise to serious problems in the present study. Trinary pairwise MEM To examine the validity of binarizing fMRI signals, we estimated the accuracy of fit of the trinary pairwise MEM as follows: First, we discretized the fMRI signal at each brain region i and each time t into one of the three different levels by thresholding. The discretized activity σ i t is set to 1, 0 and −1 if the fMRI signal was larger than ɛ , between − ɛ and ɛ and smaller than − ɛ , respectively. Then, we fitted the trinary pairwise MEM in the almost same manner as that for fitting the binary pairwise MEM [46] . Conventional FC As a control of the functional interaction, we calculated the FC based on the Pearson’s correlation coefficient between the activity of every pair of regions included in the DMN or FPN. The calculation procedures were the same as those used in previous studies of the resting-state FC [25] , [26] . After calculating the FC for each scanning session and each participant, we carried out Fisher’s transformation [28] and averaged the Z -value-based FC across sessions and participants. As is consistent with a previous study [60] , the FC matrices for the DMN and FPN were similar across participants as well as sessions for our data: Pearson’s correlation coefficient between an arbitrary pair of the FC matrices of possibly different participants and sections was >0.81. The large correlation values suggest that the averaged FC is a good representation of the FC for a single participant and session. Inverse Gaussian model As another control, we estimated functional interaction using the inverse Gaussian model. In this model, the probability density function of the brain activity is assumed to obey the multivariate Gaussian distribution given by , where X t =[ X 1 ( t ), X 2 ( t ),… X N ( t )] is the N -dimensional row vector representing the continuous-valued activity at the N regions at time t , is the row vector of the activity at the N regions averaged over sessions and participants, and is the N × N covariance matrix. In this model, we define the interaction weight between regions i and j as the ( i , j ) element of matrix Γ −1 . Partial correlation method As another control, we estimated functional interactions using the partial correlation method [36] , [37] . Using the inverse of the covariance matrix, we defined the partial correlation between brain regions i and j , denoted by r ij , by . MI method As another control, we estimated functional interactions using the MI method. In accordance with the previous studies [37] , [38] , [39] , we first estimated the MI between regions i and j at frequency ω k by , where mCoh ij ( ω k ) represents the multiple coherence between fMRI signals at regions i and j at frequency ω k [37] . We then obtained the MI between i and j , MI ij , by averaging MI ij ( ω k ) over ω k (0.01 Hz≤ ω k ≤0.1 Hz). Comparison with anatomical connexions We used the anatomical connexions among the regions in the DMN and FPN that are determined by a previous DTI study employing 80 healthy young adults [42] . In the study [44] , the authors obtained the DTI data in a Siemens Sonata 1.5T MRI scanner (Siemens Medical Systems, Germany) by using a twice-refocused single-shot Echo-Planar Imaging-based sequence (3 mm slice thickness with no inter-slice gap, 40 axial slices, TR=6,400 ms, TE=88 ms, 6 diffusion directions). The DTI data were preprocessed in SPM5 and mapped to a template of ICBM 152 in the Montreal Neurological Institution space. The anatomical connexions were determined with the use of DTI deterministic tractography. We classified the estimated values of the interaction weights between region pairs into a group of anatomically connected pairs and a group of anatomically unconnected pairs. We compared the two groups by using the two-sample t -test. As the anatomical connexions observed in DTI do not distinguish excitatory and inhibitory interactions, we submitted absolute values of the estimated interaction weights to the t -test. However, for the FC, we also submitted the raw FC values to the t -test, as was done in previous reports [34] . By conducting the ROC analysis, we obtained the accuracy with which the magnitude of the interaction weight predicts the presence and absence of the anatomical connexions. We drew ROC curves by plotting the true positive (that is, anatomically connected pairs whose interaction weights exceed a threshold) against the false positive (that is, anatomically unconnected pairs whose interaction weights exceed the same threshold) for various values of the classification threshold. For an ROC curve, the AUC is equal to the area below the ROC curve and represents the classification accuracy of the estimation method [34] . The deviation of the AUC was estimated based on a bootstrap method. How to cite this article: Watanabe, T. et al. A pairwise maximum entropy model accurately describes resting-state human brain networks. Nat. Commun. 4:1370 doi: 10.1038/ncomms2388 (2013).